Demonstration of a low-frequency three-dimensional terahertz bullet with extreme brightness The brightness of a light source defines its applicability to nonlinear phenomena in science. Bright low-frequency terahertz (<5 THz) radiation confined to a diffraction-limited spot size is a present hurdle because of the broad bandwidth and long wavelengths associated with terahertz (THz) pulses and because of the lack of THz wavefront correctors. Here using a present-technology system, we employ a wavefront manipulation concept with focusing optimization leading to spatio-temporal confinement of THz energy at its physical limits to the least possible three-dimensional light bullet volume of wavelength-cubic. Our scheme relies on finding the optimum settings of pump wavefront curvature and post generation beam divergence. This leads to a regime of extremely bright PW m −2 level THz radiation with peak fields up to 8.3 GV m −1 and 27.7 T surpassing by far any other system. The presented results are foreseen to have a great impact on nonlinear THz applications in different science disciplines. Brightness defines a light source’s ability to nonlinearly interact with matter by driving it out of an equilibrium state. Qualitatively, the brightness reveals the power concentrated at a given frequency in a solid angle according to P / λ 2 , where P and λ are the total power and wavelength. The Rayleigh criterion defines a fundamental limit for a source brightness as it correlates the minimum achievable spot size to a given λ , known as the diffraction limit. To approach this ultimate limit experimentally, an excellent source beam quality and carefully designed beam imaging optics are required. In laser physics, the quality factor M 2 is commonly used to describe how much the beam quality of monochromatic radiation deteriorates from the ideal diffraction-limited case. A high-quality beam ( M 2 ≈1) of ultrabroadband radiation is hard to achieve even for mature laser technology at near infrared wavelengths. At terahertz (THz) frequencies (0.1–10 THz), beam quality and brightness are peculiar hurdles for several reasons. First, the THz generation efficiency and the resulting pulse energy are low. Second, high brightness is by nature harder to achieve for THz than it is for radiation at shorter wavelengths. For example, for a given power, the maximum brightness of a single-cycle laser pulse at 1 THz is five orders of magnitude lower than its equivalent at a typical near infrared frequency (300 THz) exploiting the 1/ λ 2 dependence. Finally, beam imaging and focusing of multi-octave spanning THz pulses are demanding and less-developed than for other wavelength ranges [1] . Recently, the advance of intense THz sources towards ≈0.1 GV m −1 field strength enabled first observations of nonlinear light matter interactions [2] , [3] , [4] , [5] , [6] , the induction of insulator-to-metal transitions [7] and the cause of DNA damage [8] . However, a large range of THz applications, ranging from ultrafast domain switching [9] , [10] , [11] to particle acceleration [12] , requires a giant leap in brightness to match the theoretically predicted needs in field strength being on the order of a few GV m −1 . Intense THz radiation is mainly generated by employing electron accelerators [13] , [14] , [15] and laser-based systems. Although the former has been ahead in terms of intensity, the availability and versatility of lasers are dominating time-resolved THz high-field science. The most prominent techniques for intense THz pulse generation, by employing a femtosecond amplified laser pulse, are based on laser-driven ion acceleration [16] , emission from a gas plasma [17] and optical rectification in inorganic (for example, LiNbO 3 ) [18] and organic nonlinear crystals (for example, 2-(3-(4-hydroxystyryl)-5,5-dimethylcyclohex-2-enylidene)malononitrile) (OH1), 4- N,N -dimethylamino-4′- N ′-methyl-stilbazolium tosylate (DAST), 4- N,N -dimethylamino-4′- N ′-methyl-stilbazolium 2,4,6-trimethylbenzenesulfonate (DSTMS)) [19] , [20] , [21] . So far, the peak fields from these systems have been limited to 0.12–0.5 GV m −1 . In ref. 22 , a peak electric field of 10.8 GV m −1 was reported from difference frequency generation. However, at such intensity, the carrier frequency was 30 THz, which is beyond the range commonly associated with THz frequencies (0.1–10 THz). Compact laser-based LiNbO 3 THz sources deliver currently the largest pulse energy (125 μJ) [23] but it needs a non-collinear pump configuration with sophisticated pulse front tilting to achieve phase matching. The maximum reported field using LiNbO 3 was demonstrated at significantly lower pulse energy (3 μJ) only. This is a direct consequence of shortened THz beam quality induced by such a non-collinear pumping scheme, which makes diffraction-limited focusing a challenge. Much brighter radiation is expected from collinearly pumped THz schemes as the THz pulse front is untilted and the intensity profile is expected to be similar to the pump profile. In this report, using a conventional and collinear THz generation scheme based on optical rectification in the small-size, highly efficient organic crystals DSTMS and OH1, we present a concept based on pump-pulse divergence control where the THz wavefront and imaging is engineered to reach the ultimate confinement of a THz pulse in the λ 3 volume. The process is accompanied by significant upscaling of the THz intensities. We observed the beam propagating in this so-called lambda-cubic regime to significantly alter the temporal and spectral characteristics along the propagation axis in the focus. For our THz source, we use an optical parametric amplifier (OPA) system with pulse duration of 65 fs to pump small-size organic crystals DSTMS and OH1 at 1.5 and 1.35 μm wavelengths (see Methods for more details). In our scheme, an all-reflective telescope assembly is used to adapt the spherical wavefront curvature of the pump beam at the position of the THz emitting organic crystal where the pump fluence is kept constant. The organic crystals are excellently suited for THz generation as they offer phase-matched THz generation in the 1–5 THz range (where no inorganic crystal was proven efficient), a very high second-order nonlinear optical susceptibility (214 (ref. 24 ) and 240 pm V −1 (ref. 25 )) and high damage threshold (see Methods section for more details). Terahertz characterization Although efficient THz energy extraction from organic crystals has previously been reported [19] , [20] , the advance of the present work is the introduction of an effective scheme for enhanced THz wavefront and beam profile control and improved THz beam transport of the multi-octave spanning THz radiation, which compensates for aberrations originating from the source and from THz imaging optics. 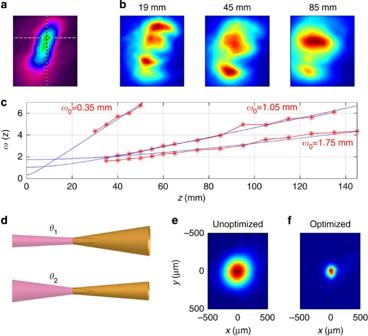Figure 1: Terahertz wavefront correction. (a) The optical pump spatial profile measured with a pyroelectric camera. The locus of the peak intensity is marked with dashed lines. (b) The spatial evolution of the generated THz profile, taken with an uncooled microbolometer array. The images are sized 5.5 × 7.3 mm2. The noted positions are measured from the emission plane. (c) Measurement of the divergence of THz emitters with variable sizes (red). The theoretical estimation is shown in blue. (d) A demonstration of the effect of optical pump convergence (pink) on the generated THz pump wavefront (golden). Bending the optical pump divergence angleθ1toθ2leads to a reduction of the generated THz divergence. The output THz pulse after focusing, (e) before and (f) after optimization. The final focusing mirrors in both systems have similar numerical apertures. Figure 1a,b shows the spatial profiles of the optical pump and the generated THz after the DSTMS crystal. The spatial profile of the pump is directly reflected in the emitted THz. Our single-crystal THz source mimics several emitters of irregular shapes and sizes. This is a direct consequence of the typically irregular thin organic crystal and the strong non-uniformity of the optical pump ( Fig. 1a , note that non-uniform intensity profiles are rather typical for high-energy OPAs). The spatial pump irregularities are more pronounced in the THz spatial profile because the THz intensity scales with the square of the pump intensity, as illustrated in Fig. 1b . Presently, there is neither an existing THz wavefront corrector nor a way to directly measure the THz wavefront. In the optimization scheme, we exploit the fact that, in the first order, wavefront and divergence are related. At a distance z from the generation crystal, the radius of curvature of the wavefront is given by z [1+( ω /( θz )) 2 ], where ω and θ are the spot size and divergence, respectively, whereas the Gaussian beam divergence is given by θ = λ /π ω with λ being the wavelength. Although a point source THz emitter exhibits a spherical wavefront (that is, strong divergence), a large-area emitter provides a close to planar wavefront (weak divergence). Ideally, for tightest focusing, one aims for a planar, frequency-independent THz wavefront right at the final focusing mirror. Because of the irregular pump intensity profile and local crystal in-homogeneities, the THz source studied here, however, mimics a superposition of several emitting zones embodying non-uniform intensity distribution with different divergence, and beam propagation properties. As illustrated in Fig. 1b , the evolution of the THz beam intensity behind the organic crystal resembles the propagation of modes of different size, shape and divergence, which leads to a change of the THz beam profile upon propagation. Far from the source, high-frequency irregularities from smaller emission spots wash out due to larger divergence, which results in a more regular intensity shape. The aforementioned qualitative picture is supported by measuring the THz divergence from different emitting zones of variable size ( ω 0 =0.35, 1.05 and 1.75 mm, respectively) in Fig. 1c , and good agreement is found with the divergence calculated from the pump spot size for a centre frequency of 2 THz (ref. 19 ). However, as the divergence angle depends on the THz frequency for a given spot size, the spectral dependence of the divergence adds additional variations to the net intensity profile. Owing to these complex beam characteristics, a perfect focusing to the lambda-cubic volume for all frequencies (that is, more than 7 octaves) emitted by our source requires an iterative optimization procedure for divergence and source position as well as the optimization of the final focusing stage. The long wavelengths associated with the THz frequencies and the multi-octave spanning frequency content poses additional hurdles as large aperture optics are required. Confining the THz energy of such a THz beam in a lambda-cubic volume for all frequencies is therefore a great challenge. Figure 1: Terahertz wavefront correction. ( a ) The optical pump spatial profile measured with a pyroelectric camera. The locus of the peak intensity is marked with dashed lines. ( b ) The spatial evolution of the generated THz profile, taken with an uncooled microbolometer array. The images are sized 5.5 × 7.3 mm 2 . The noted positions are measured from the emission plane. ( c ) Measurement of the divergence of THz emitters with variable sizes (red). The theoretical estimation is shown in blue. ( d ) A demonstration of the effect of optical pump convergence (pink) on the generated THz pump wavefront (golden). Bending the optical pump divergence angle θ 1 to θ 2 leads to a reduction of the generated THz divergence. The output THz pulse after focusing, ( e ) before and ( f ) after optimization. The final focusing mirrors in both systems have similar numerical apertures. Full size image Wavefront correction and focusing In principle, a planar wavefront could be achieved by placing the focusing optics far from the emitter. However, this leads to significant loss of the THz energy on a finite focusing optics, which is accompanied by aberrations due to spatially filtering. We therefore follow the approach of wavefront manipulation by divergence control discussed above to correct the THz wavefront from the emitter directly. As illustrated in Fig. 1d , a bending of the optical pump wavefront leads to a bending of the generated THz wavefront [26] . For a specific frequency and single emitting spot size, there is an optimum value for such a bending that compensates for the natural divergence of the emitted THz beam, thus leading to a collimated THz beam at the input of the focusing system. The procedure is combined with fast expansion of the THz beam in order to smear out the high-frequency intensity modulations. We employed low f-number optics (using a 1:4 telescope based on 1′′ and 2′′-diameter off-axis parabolic mirrors) to reduce the inevitable aberrations in the unoptimized spectral components. However, with the ultra-broad spectrum and existence of multiple emitters of different divergence at the source, only a compromise can be experimentally found for best achievable focus spot size. In order to reach the λ 3 light bullet, we systematically adjusted the pump beam wavefront curvature and the THz generation plane (crystal position) to optimize the THz peak field and spot size. This surprisingly simple approach is used to reach the physical limits of THz focusing after a few iterations, which results in a dramatic increase of the THz brightness and intensity. In order to demonstrate the advance of our approach, we compare the THz spot size before ( Fig. 1e ) and after ( Fig. 1f ) optimizing the system. The spot size is four times smaller than what was previously achieved using a non-lambda-cubic focusing scheme [19] . It is worth mentioning that the pump wavefront corrections do not compensate only for the divergence of the THz beam, but also for the low-order wavefront aberration of the subsequent focusing system. Output pulse characteristics The temporal traces of the generated pulses in the focal waist are retrieved by air-biased coherent detection (ABCD) [27] and are shown in Fig. 2a for DSTMS and OH1. Peak fields of 8.3 GV m −1 (27.7 T) and 6.2 GV m −1 (20.7 T) are achieved, respectively. The absolute electric field strengths are obtained in a model-independent way, by measuring the THz pulse energy, spot size and the temporal field evolution. In the lambda-cubic regime presented here, we observe that the measured single-cycle carrier oscillates faster than previously reported from an identical DSTMS [19] (with similar pump-pulse duration and crystal thickness). Furthermore, we observe a high-frequency amplitude modulation in the temporal trace of OH1. These observations are a direct consequence of the improved beam quality and tight focusing scheme where high-frequency THz components get dominant in the beam waist at the diffraction limit. Such high-frequency features were observed even with electro-optical sampling (EOS) detection as we show in the Methods section. The spectral amplitudes are given in Fig. 2b showing THz emission between 0.1 and 12 THz. More details on the spectral features are given in the Methods section. We measured the THz spot size ( Fig. 2c,d ) using an uncooled pyroelectric array detector (NEC Inc., 23.5 μm pixel size). After optimization of wavefront and focusing, the average radii at 1/ e 2 were 70 and 59 μm from DSTMS and OH1. When we used an off-axis mirror with a hole (to pass the probe beam), the spot sizes were slightly larger (93, and 70 μm) as shown in Fig. 2e,f . The measured spot sizes are strikingly small under consideration of the spectra from these crystals. Thanks to wavefront control, the THz spot size is more than four times smaller than in previous reports (300 μm) [19] using the same crystal DSTMS and similar input beam size. This tight focusing enhances the THz peak intensity by more than an order of magnitude. 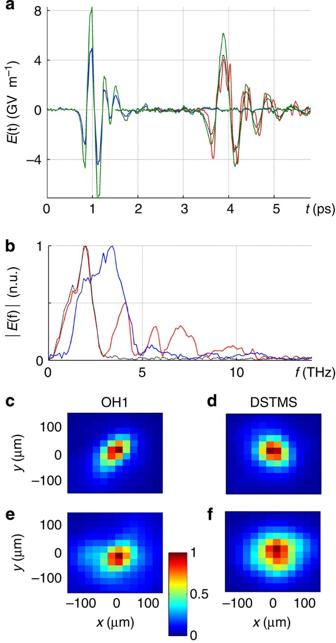Figure 2: The characteristics of the generated pulses. (a) The temporal profiles of the THz pulses generated from DSTMS (blue) and OH1 (red and shifted in time). The black curve shows the corresponding temporal profile from OH1 after removing the high-frequency modulations using a 3 THz low-pass filter. The green curves show the estimated THz profile for a focusing mirror without probe hole. The peak fields reach 8.3 GV m−1(27.7 T) and 6.2 GV m−1(20.7 T) from the two crystals, respectively. (b) The corresponding THz amplitude spectra. The THz spot at the detector using a focusing mirror without a probe hole from (c) OH1 and (d) DSTMS, measured with a THz camera and shown in normalized units. (e,f) The corresponding spots when we used a holey mirror for THz focusing. Figure 2: The characteristics of the generated pulses. ( a ) The temporal profiles of the THz pulses generated from DSTMS (blue) and OH1 (red and shifted in time). The black curve shows the corresponding temporal profile from OH1 after removing the high-frequency modulations using a 3 THz low-pass filter. The green curves show the estimated THz profile for a focusing mirror without probe hole. The peak fields reach 8.3 GV m −1 (27.7 T) and 6.2 GV m −1 (20.7 T) from the two crystals, respectively. ( b ) The corresponding THz amplitude spectra. The THz spot at the detector using a focusing mirror without a probe hole from ( c ) OH1 and ( d ) DSTMS, measured with a THz camera and shown in normalized units. ( e , f ) The corresponding spots when we used a holey mirror for THz focusing. Full size image Temporal and spectral modulation around the focus In lambda-cubic focusing, the temporal and spectral shapes of the THz are expected to alter rapidly across the waist as the Rayleigh length is minimized. In Fig. 3a,b , we show time domain maps of the THz temporal profile from DSTMS and OH1, respectively, reconstructed in the propagation ( z ) direction around the focus position ( z = z 0 ). It illustrates the Gouy phase shift of π across ( z − z 0 ) >>| z R | with z R being the Rayleigh length. 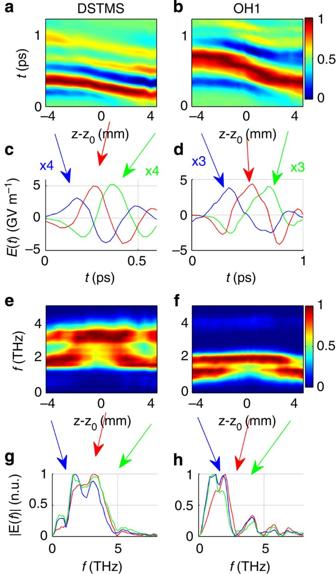Figure 3: Temporal and spectral modulation around the focus. Two-dimensional (normalized) maps of the THz time traces across the focus in the case of (a) DSTMS and (b) OH1, constructed with EOS detection. (c,d) Visualization of the Guoy effect across the focus with traces taken fromaandb. (e,f) Two-dimensional maps of the normalized THz spectra versus position showing the shift of the spectrum centre across the THz focus.z0is the position of the focal plane. (g,h) The corresponding spectra of the time traces incandd. Figure 3c,d illustrates the temporal field evolution at positions ( z − z 0 )={−4, 0, 4} mm and the fast decay of field strength for | z |>0. The spectral evolution across the waist ( Fig. 3e–h ) shows a strong shift of the centre frequency towards higher frequencies as we approach the focus position. This is a direct consequence of the λ 3 focusing scheme where the linear dependence of the spot size ω 0 on the THz wavelength is highly pronounced as the λ 3 volume for lower frequencies is larger. These results contrast a recent report for THz focusing at (loose) non-λ 3 conditions. Under the latter condition, the spectrum is experimentally found to get broader around the focus with no shift in the centre [19] . Figure 3: Temporal and spectral modulation around the focus. Two-dimensional (normalized) maps of the THz time traces across the focus in the case of ( a ) DSTMS and ( b ) OH1, constructed with EOS detection. ( c , d ) Visualization of the Guoy effect across the focus with traces taken from a and b . ( e , f ) Two-dimensional maps of the normalized THz spectra versus position showing the shift of the spectrum centre across the THz focus. z 0 is the position of the focal plane. ( g , h ) The corresponding spectra of the time traces in c and d . Full size image Beam quality and diffraction-limited focusing Evaluation of the beam quality parameter M 2 requires three-dimensional beam profiling around the focus. As the THz radiation covers several octaves, the spectrum is added as a fourth dimension. We did time domain spectroscopy along the beam propagation direction across the focus using EOS detection. Then, we evaluated z R from the corresponding decrease in the axial beam intensity ( Fig. 4a ). From this, we obtained both the spot size ( Fig. 4b ) and an effective numerical aperture (NA; Fig. 4c ). This technique neglects the effect of the detector and assumes a highly symmetric Gaussian beam. In our case, it overestimates z R because of the overall large probe size that is nearly collimated along the scanned beam waist. Our experimental estimation of the effective NA was then compared against the NA calculated assuming a high-quality diffraction-limited ( M 2 =1) beam. The good matching suggests that our beam has M 2 ≈1 within a slight frequency dependence arising from the minimized-but-unavoidable divergence and imperfections in both the optical pump and generating crystals. 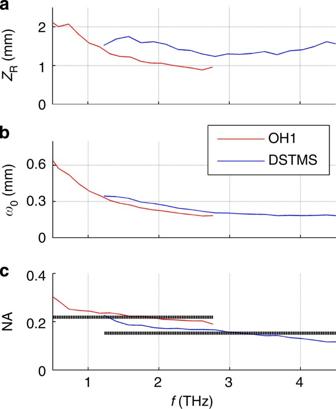Figure 4: Beam quality and diffraction-limited focusing. (a) Rayleigh length, (b) minimum focus size and (c) the effective numerical aperture estimated from the spot size. The solid lines show the calculated numerical aperture assuming a diffraction-limited system with quality factorM2=1. Figure 4: Beam quality and diffraction-limited focusing. ( a ) Rayleigh length, ( b ) minimum focus size and ( c ) the effective numerical aperture estimated from the spot size. The solid lines show the calculated numerical aperture assuming a diffraction-limited system with quality factor M 2 =1. Full size image In a lambda-cubic focusing scheme, the focus volume depends strongly on the THz frequency. 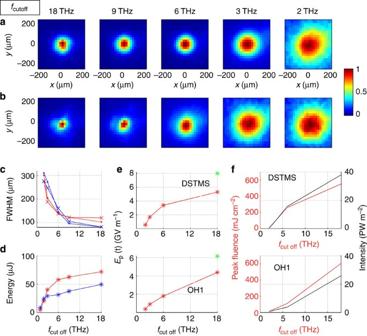Figure 5: Spot size and field and intensity characterization. The normalized THz spot at the focus is shown for (a) DSTMS and (b) OH1 for different cut off frequencies {2,3,6,9,18} THz. (c) The extracted THz spot size at full-width-half-maximum fromaandbfor different cut off frequencies. Red and blue refer to DSTMS and OH1, respectively. The dot and cross markers denote thexandydirections. (d) The corresponding energies for DSTMS (red) and OH1 (blue). (e) The THz peak electric fields. (f) The measured peak fluence and peak intensities. Ine, the green asterisks denote the estimated field when a focusing mirror without a probe hole was used. Apart from this, all the measurement were taken with a holey focusing mirror. Figure 5 illustrates this lambda-cubic dependence of the intensity in the focus. A set of low-pass filters (LPFs) is used to measure the evolution of the spot size with frequency. As expected there is a monotonic decrease of the spot size for higher THz components. This is a consequence of the tight focusing where the intensities of the high-frequency components go up dramatically dominating the contribution of the low-frequency components to the overall imaged spot size. Although the two crystals show a similar trend for radiation <2 THz, its evolution with frequency is quite different ( Fig. 5a,b ). In the case of DSTMS, ω 0 drops significantly for cutoffs at 3 and 6 THz, followed by bare change for a further increase in the cutoff frequency. This implies that the majority of the energy is concentrated at low frequencies ( Fig. 5c ), which is in line with the ABCD measurements shown in Fig. 2 . In contrast, OH1 shows a much broader distribution of energy, especially in the 6–9 THz range. We measured the corresponding energy using a calibrated Golay cell (which has almost frequency-independent response in our spectral range). The above-predicted energy buildup rate with frequency from the two crystals is well demonstrated in Fig. 5d . The total energy measured was 109 μJ from DSTMS and 76 μJ from OH1 (without holey mirror losses) at pump energies of 3.8 and 3.5 mJ, respectively. The corresponding conversion efficiencies are 2.86% and 2.14%, respectively. The energy losses on the holey mirror were around 30% because of the large hole size required for ABCD detection. Figure 5: Spot size and field and intensity characterization. The normalized THz spot at the focus is shown for ( a ) DSTMS and ( b ) OH1 for different cut off frequencies {2,3,6,9,18} THz. ( c ) The extracted THz spot size at full-width-half-maximum from a and b for different cut off frequencies. Red and blue refer to DSTMS and OH1, respectively. The dot and cross markers denote the x and y directions. ( d ) The corresponding energies for DSTMS (red) and OH1 (blue). ( e ) The THz peak electric fields. ( f ) The measured peak fluence and peak intensities. In e , the green asterisks denote the estimated field when a focusing mirror without a probe hole was used. Apart from this, all the measurement were taken with a holey focusing mirror. Full size image We measured peak electric fields of 5.4 GV m −1 (17.8 T) and 4.4 GV m −1 (14.7 T) from DSTMS and OH1, respectively ( Fig. 4e ). These values were obtained from small aperture organic crystals, in comparison with 0.5 GV m −1 obtained from a large aperture DSTMS [20] . Figure 4e shows the obtained peak fields when LPF with different cutoff frequencies were used. Higher frequency components correspond to short pulse duration and, in our case, to small spot size as well. This, in turns, leads to higher field intensities ( Fig. 5e ). We estimated the peak fluence and intensity to be {552, 610} mJ cm −2 and {38, 26} PW m −2 for DSTMS and OH1, respectively ( Fig. 5f ). Finally, the presented results considered the whole spectral range up to 18 THz. However, from DSTMS most of the energy is concentrated in the 1–5 THz, which we consider the most important part of this work. In the sub-5 THz range, high-peak field (3.4 GV m −1 , 11.4 T), peak fluence (260 mJ cm −2 ) and peak intensities (15.7 PW m −2 ) are achieved using DSTMS, which are the highest ever reported values in the whole THz band so far. If we take into account the losses due to the usage of the holey mirror (which is not required for non-collinear probe experiments [2] ), the peak field from DSTMS is 8.3 GV m −1 (27.7 T) and peak intensity is 110 PW m −2 . At the extreme peak fields reported here, even THz-induced ionization and damage could occur. Combining such intensities with field enhancement structures [7] , [28] , [29] will lead to another giant leap in intensities. In conclusion, we have experimentally presented a λ 3 THz bullet using low-frequency ultrabroadband THz pulses. Our result is perhaps the first demonstration of such a system in the entire electromagnetic spectrum. This approach allowed us to reach, by far, the most intense low-frequency THz pulses between 1–5 THz (DSTMS) and up to 18 THz (OH1). Our work introduces a concept based on pump wavefront-divergence control combined with an improved imaging scheme to significantly enhance the THz beam quality and THz brightness in a collinear pump scheme based on a small-scale organic crystal. The method leads to extremely intense THz radiation of 110 PW m −2 and field strength of 8.3 GV m −1 and 27.7 T. Such a compact ultra-intense THz source with such an extreme brightness will open up new avenues for nonlinear THz applications in a wide range of science. Terahertz generation system Our THz source consists of a 100-Hz Ti-Sapphire-driven three-stage OPA system with pulse duration around 65±5 fs. This source is used to pump small-size organic crystals at 1.5 μm for DSTMS (thickness of 440 μm and diameter of 6 mm) and 1.35 μm for OH1 (thickness of 480 μm and diameter of 10 mm). The overall OPA conversion efficiency is ~39%. Taking beam transmission losses into account, pump energies of 3.8 and 3.5 mJ are available for pumping the nonlinear crystal, at the two respective wavelengths. The measurements presented here have been done at the maximum energies. The spot size of the pump beam on the crystal had 1/ e 2 dimensions of 3.8 and 4.1 mm, respectively, corresponding to a peak fluence of ~23 mJ cm −2 . This is close to the crystals’ damage threshold. The crystal’s cut and orientation was chosen for the maximum THz generation, following refs 24 , 25 . 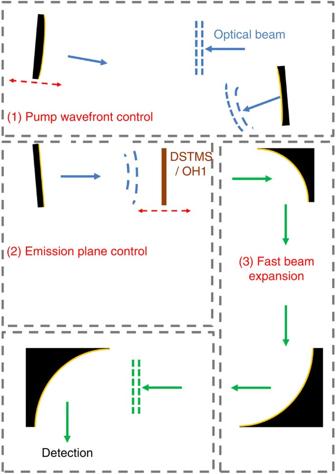Figure 6: Focusing optimization schematic. The three stages of optimization are marked with red on the schematic. Figure 6 shows a schematic diagram of the THz setup with the three main optimization stages: (i) pump wavefront control stage where a reflective telescope is used to bend the pump-pulse wavefront by means of readjusting the spacing between the two mirrors of the telescope, (ii) THz generation where the THz emission plane (crystal position) is adjusted along with the first stage for an optimum focusing and (iii) fast expansion of the beam using parabolic mirrors. The fast expansion helps minimize the effect of the natural divergence in the generated beam and thus better control over the THz wavefront. The resulting nearly planar wavefront beam is thus focused on the detector using 2′′-diameter, 2′′-focal distance off-axis mirror. To attenuate the THz beam, we used a set of 400-μm-thick Silicon wafers (each having almost frequency-independent amplitude transmission of 70%). To block the residual OPA beam after the generation crystal, we used three LPF with cutoff frequency of 18 THz with an out-of-band blocking better than 0.1% each. Figure 6: Focusing optimization schematic. The three stages of optimization are marked with red on the schematic. Full size image Spectral features of the generated THz pulses The THz spectra produced by optical rectification in nonlinear crystals depend on the effective generation crystal length and the pump spectrum. For a transform-limited 65 fs pump pulse (full-width at half-maximum)), the ideal THz spectrum should reflect an optically rectified spectrum centred around 5.7 THz with a full-width at half-maximum of 9.5 THz (ref. 30 ). However, DSTMS and OH1 (as most of the THz generating crystals) have strong phonon absorptions in this range that significantly modulate the spectrum. The amplitude spectra of THz pulses produced in DSTMS and OH1 are shown in Fig. 2b . The strong features in the spectra reflect the phonon resonance in this region. DSTMS has a strong absorption resonance at 1.024 THz. In the 1–4 THz range, there are no strong resonances [25] . We did not find data on resonances/linear characterization beyond 4 THz, but we observed a strong absorption around 4.9 THz, which likely comes from another resonance ( Fig. 2 ). OH1 shows a higher spectral density at lower frequency going along with a wider spread of spectral density at least up to 12 THz. The main absorption resonances occur at 1.45 and 2.85 THz (consistent with previous reports [26] ). Here again we could not find reports on higher frequencies resonances, but from our spectrum we anticipate resonances around {4.9, 6.3} THz. In the section ‘output pulse characteristics’, we drew a comparison with ref. 19 . Note that although the f-number of the detector focusing mirror in our measurement is different from ref. 19 , the NA of the main spectral contents was nearly the same as discussed in the article. Spot size imaging and calibration To image the THz spot size, we used a microbolometer camera from NEC Inc. It is currently the most sensitive THz sensor on the market. However, the manufacturer states that the frequency range is 1–7 THz and is based on evaluation and calculated results with no guarantee due to the lack of a standard calibration method. We are unaware of any report of it being used at such high frequencies. In the estimation of the peak field from the measured energy, we considered the energy and the pulse duration of the main lobe (half cycle with peak field) of the pulse. Intensity calculations were performed following ref. 31 . Terahertz detection Throughout this work, we used two different detections schemes: ABCD and EOS. For EOS, we used a GaP crystal with thickness of 100 μm. We compared the time trace with that from a 50 μm and got the same trace but we used the thicker one in order to avoid the internal reflection. A comparison between the measured pulses from the two techniques is shown in Fig. 7 . 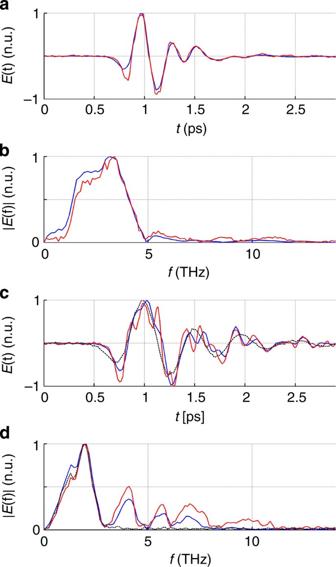Figure 7: Terahertz detection schemes. A comparison between the measured THz from DSTMS (a,b) and OH1 (c,d). The blue curves show the measurement using EOS. Air-biased coherent detection measurements are shown in red. In the case of OH1, another measurement (black) was taken with ABCD after filtering out the higher frequency (>3 THz) components. Figure 7: Terahertz detection schemes. A comparison between the measured THz from DSTMS ( a , b ) and OH1 ( c , d ). The blue curves show the measurement using EOS. Air-biased coherent detection measurements are shown in red. In the case of OH1, another measurement (black) was taken with ABCD after filtering out the higher frequency (>3 THz) components. Full size image How to cite this article: Shalaby, M. and Hauri, C. P. Demonstration of a low-frequency three-dimensional terahertz bullet with extreme brightness. Nat. Commun. 6:5976 doi: 10.1038/ncomms6976 (2015).